Diversity-oriented synthesis as a tool for identifying new modulators of mitosis The synthesis of diverse three-dimensional libraries has become of paramount importance for obtaining better leads for drug discovery. Such libraries are predicted to fare better than traditional compound collections in phenotypic screens and against difficult targets. Herein we report the diversity-oriented synthesis of a compound library using rhodium carbenoid chemistry to access structurally diverse three-dimensional molecules and show that they access biologically relevant areas of chemical space using cheminformatic analysis. High-content screening of this library for antimitotic activity followed by chemical modification identified ‘Dosabulin’, which causes mitotic arrest and cancer cell death by apoptosis. Its mechanism of action is determined to be microtubule depolymerization, and the compound is shown to not significantly affect vinblastine binding to tubulin; however, experiments suggest binding to a site vicinal or allosteric to Colchicine. This work validates the combination of diversity-oriented synthesis and phenotypic screening as a strategy for the discovery of biologically relevant chemical entities. Diversity-oriented synthesis (DOS) aims to synthesize libraries of structurally complex and functionally diverse small molecules in an efficient manner [1] , [2] . Biomolecules interact with each other in a three-dimensional environment and, consequently, functional diversity is directly associated with the three-dimensional chemical information the surface of a small molecule presents when interacting with macromolecules, such as proteins. The last decade has witnessed the emergence of several distinct DOS strategies for the construction of chemically diverse libraries [3] , [4] , [5] . One such method, the reagent-based approach [3] , involves synthesizing one or more densely functionalized molecules, which can subsequently be transformed into diverse molecular scaffolds. These molecules can be reacted selectively with a wide variety of reagents, providing access to an array of distinct molecular frameworks. Alternatively, a single pluripotent functional group can be exploited by subjecting it to a wide variety of reaction conditions, thereby enabling the synthesis of multiple molecular skeletons. Carbenoid chemistry offers exciting opportunities for DOS applications, particularly in the context of the reagent-based approach. A wealth of distinct reactions can be performed using carbenoid chemistry [6] , and its applicability to library construction was recently exemplified by Panek and coworkers [7] . In addition to scaffold diversity, increasing the carbogenic sp 3 content and the number of stereocentres has been suggested to enhance the selectivity and potency for a given target, and increase the hit rate across several targets from a single library [8] . Furthermore, increasing sp 3 count correlates favorably with decreasing clinical toxicity [9] , and decreasing aromatic ring count is likely to produce less compound attrition in drug discovery [10] . It is important that these considerations are implemented in DOS strategies, and that effective methods are developed to enable the efficient synthesis of structurally diverse compound collections. Phenotypic screening is an expedient approach for identifying small molecules that perturb biological function. It provides an efficient way to evaluate the biological activity of a compound collection against a wide variety of molecular targets [11] . Recently, it has also been established that the vast majority of first-in-class drugs were identified by phenotypic screening [12] . Our group and others have successfully implemented this approach in combination with DOS to discover novel small-molecule modulators of biological function [13] . In 2008, we discovered gemmacin, a small molecule with similar potency to clinically used antibiotics and improved activity against resistant bacterial strains [14] . Other groups have also used this approach effectively; some notable examples include the discovery of the novel Hedgehog pathway modulator robotnikinin [15] , and compounds with interesting antimalarial properties [16] . Another related approach, termed biology-oriented synthesis, has also led to the identification of many useful tool compounds from phenotypic screens [17] , [18] , [19] . Phenotypic screening has been used effectively to discover new antimitotics [20] , [21] . While several clinically used antimitotics exist, they often suffer from administration or resistance problems [22] , [23] . Additionally, they are mostly derived from natural products, making chemical modification difficult. Therefore, the discovery of new compounds that cause mitotic arrest is potentially important. Here we report the efficient synthesis of a functionally diverse compound collection, using rhodium carbenoid chemistry in a reagent-based approach. These molecules display a high sp 3 content and access biologically relevant areas of chemical space. Furthermore, using phenotypic high-content screening, we present the biological evaluation of these compounds using an assay detecting the induction of mitotic arrest. We present one hit series, which induces mitotic arrest by depolymerizing microtubules and binds in a site vicinal or allosteric to Colchicine. Library synthesis To synthesize the library, we developed a reagent-based DOS approach employing rhodium carbenoid chemistry to produce pluripotent substrates, from which a range of structurally diverse small molecules could be regio- and diastereo-selectively synthesized. To this end, we envisaged the use of phenyldiazo ester compounds ( 1 and 12 ) as highly functionalized substrates, from which a structurally complex compound collection could be constructed ( Figs 1 and 2 ). Rhodium-catalysed cyclopropanation of compound 1 , which was obtained according to the literature precedent [24] , with a range of unsaturated compounds led to the formation of densely functionalized molecular frameworks ( Fig. 1 ). The diastereo-selective reaction of 1 with terminal alkynes and alkenes provided cyclopropenes and cyclopropanes, respectively, in good yields and complete diastereocontrol for 4 ( Fig. 1 , pathways a and c) [25] . Cyclopropene 2 was subsequently diversified by palladium-catalyzed C–H activation, coupling 2 with p- nitroiodobenzene using Heck-type reaction conditions to yield 3 (ref. 26 ). The generation of functionality variants was accomplished by the reaction of 1 with various allenes, affording the corresponding cyclopropanes with exocyclic alkenes ( 5-6 ), which could be converted to the lactones ( 7–8 ) via iodolactonization [27] . The remaining iodide was then successfully removed by radical deiodination to give 9 and 10, completing a subset of the library based on 1 . 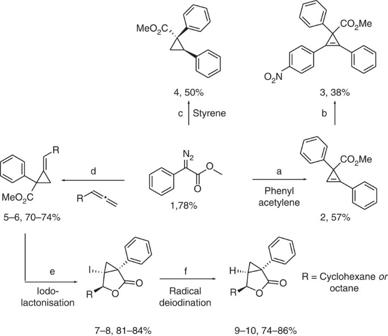Figure 1: Synthetic scheme of DOS library subset based on1. (a) Phenylacetylene, Rh2(OAc)4(1 mol%), CH2Cl2; (b)p-nitroiodobenzene, Pd(OAc)2(10 mol%), K2CO3, DMF; (c) styrene, Rh2(OAc)4(1 mol%), CH2Cl2; (d) undeca-1,2-dieneorpropa-1,2-dien-1-ylcyclohexane, Rh2(OAc)4(1 mol%), CH2Cl2; (e)N-iodosuccinimide, MeCN-H2O (2:1), 50 °C; (f) Bu3SnH, AIBN, PhH, 80 °C. Figure 1: Synthetic scheme of DOS library subset based on 1 . (a) Phenylacetylene, Rh 2 (OAc) 4 (1 mol%), CH 2 Cl 2 ; (b) p -nitroiodobenzene, Pd(OAc) 2 (10 mol%), K 2 CO 3 , DMF; (c) styrene, Rh 2 (OAc) 4 (1 mol%), CH 2 Cl 2 ; (d) undeca-1,2-diene or propa-1,2-dien-1-ylcyclohexane, Rh 2 (OAc) 4 (1 mol%), CH 2 Cl 2 ; (e) N- iodosuccinimide, MeCN-H 2 O (2:1), 50 °C; (f) Bu 3 SnH, AIBN, PhH, 80 °C. 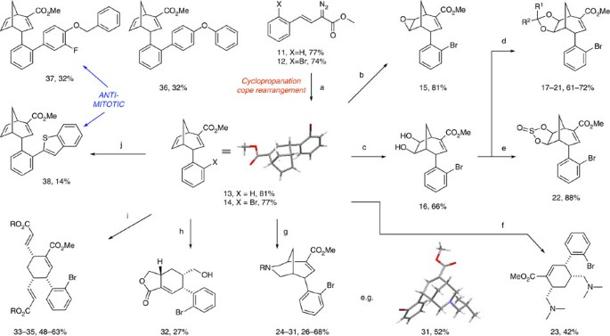Figure 2: Library synthesis from key building block14. (a) Cyclopentadiene, Rh2(OAc)4(1 mol%), CH2Cl2; (b)m-CPBA, CH2Cl2; (c) OsO4(2.5 mol%), NMO, acetone-H2O (9:1); (d) aldehyde/ketone, CSA (10 mol%), 3 Å molecular sieves, CH2Cl2; (e) SOCl2, CH2Cl2; (f) 2,6-lutidine, NMO, OsO4(2.5 mol%), PhI(OAc)2, acetone-H2O (10:1), then dimethylamine, NaBH(OAc)3, CH2Cl2; (g) 2,6-lutidine, NMO, OsO4(2.5 mol%), PhI(OAc)2, acetone-H2O (10:1), then primary amine, NaBH(OAc)3, CH2Cl2; (h) 2,6-lutidine, NMO, OsO4(2.5 mol%), PhI(OAc)2, acetone-H2O (10:1), then NaBH4, MeOH; (i) alkene, Hoveyda–Grubbs (II) catalyst (10 mol%), ethylene, PhMe, 100 °C; (j) Pd(OAc)2(10 mol%), PPh3(15 mol%), 2 N K2CO3, PhMe, 90 °C. Full size image Figure 2: Library synthesis from key building block 14 . (a) Cyclopentadiene, Rh 2 (OAc) 4 (1 mol%), CH 2 Cl 2 ; (b) m- CPBA, CH 2 Cl 2 ; (c) OsO 4 (2.5 mol%), NMO, acetone-H 2 O (9:1); (d) aldehyde/ketone, CSA (10 mol%), 3 Å molecular sieves, CH 2 Cl 2 ; (e) SOCl 2 , CH 2 Cl 2 ; (f) 2,6-lutidine, NMO, OsO 4 (2.5 mol%), PhI(OAc) 2 , acetone-H 2 O (10:1), then dimethylamine, NaBH(OAc) 3 , CH 2 Cl 2 ; (g) 2,6-lutidine, NMO, OsO 4 (2.5 mol%), PhI(OAc) 2 , acetone-H 2 O (10:1), then primary amine, NaBH(OAc) 3 , CH 2 Cl 2 ; (h) 2,6-lutidine, NMO, OsO 4 (2.5 mol%), PhI(OAc) 2 , acetone-H 2 O (10:1), then NaBH 4 , MeOH; (i) alkene, Hoveyda–Grubbs (II) catalyst (10 mol%), ethylene, PhMe, 100 °C; (j) Pd(OAc) 2 (10 mol%), PPh 3 (15 mol%), 2 N K 2 CO 3 , PhMe, 90 °C. Full size image Encouraged by the scope of complexity-generating methodology accessible via the rhodium (II)-catalyzed carbenoid chemistry, we decided to synthesize the styryl diazoester derivatives 11 and 12 . Davies et al. [28] demonstrated the ability of 11 to undergo tandem cyclopropanation-cope rearrangement reactions, resulting in the diastereo-selective formation of highly functionalized bicyclo[3.2.1]octadienes. We hypothesized that the synthesis of a cycloheptadiene scaffold from a styryl diazoester containing an ortho-bromo aryl functionality (as in compound 12 ) would furnish a bicyclic construct poised for further diversification. Adorned with reactive functionality, intermediate 12 could be subjected to a variety of diversity-generating reactions, thus providing a library of skeletally diverse small molecules containing multiple stereocentres. Taking precedent from the described synthesis of 11, compound 12 was initially synthesized via the Wittig olefination of bromobenzaldehyde, followed by esterification and diazo formation ( Supplementary Fig. 1 ). However, the Wittig reaction provided a mixture of ( E ) and ( Z ) stereoisomers, presumably due to steric hindrance of the bromo substituent. Optimization of the synthetic route followed; treating 2-bromophenyl acetaldehyde with malonic acid in Hünigs base provided the Knoevenagel condensation product. Subsequent esterification delivered a mixture of regioisomers ( Supplementary Fig. 1b ), which was readily converted to the desired diazo compound 12 as a single ( E ) stereo- and regioisomer. Intermediate 12 was subjected to a cyclopropanation-cope rearrangement according to the procedure developed by Davies et al. [28] to provide the highly functionalized key intermediate 14 in good yield ( Fig. 2 ). This reaction delivered three new stereocentres with complete diastereocontrol, thereby enabling further diversification via stereocontrolled reactions. The presence of both an electron-deficient and an electron-neutral olefin in the bicyclic system, coupled with the proximal aryl bromide and a carboxylic acid ester in the backbone of compound 14, afforded the opportunity to regioselectively modify the scaffold in a multidirectional approach. Our exploration of the chemical space around scaffold 14 began with a stereoselective epoxidation reaction, resulting in the formation of epoxide 15 on the less hindered face in excellent yield. The relative stereochemistry of this compound was confirmed by nuclear overhauser effect spectroscopy (NOESY) experiments, which showed no interaction between the methine epoxide protons and those of the fused ring bridgehead. Regio- and stereoselective dihydroxylation of the electron-neutral alkene was performed under Upjohn conditions, using osmium tetroxide, thereby providing the chiral cis -diol 16 , containing five contiguous stereocentres, and a further molecular construct poised for diversification. The stereochemical relationship of the two new sterocentres confirmed that the dihydroxylation reaction occurs selectively from the less hindered face of bicyclo[3.2.1]octadiene 14 . Reacting diol 16 with commercial aldehydes and ketones under acidic conditions provided acetals 17–21 in good yield. Finally, sulfoxide 22 , which comprises six chiral centres, was readily synthesized as a 3:1 mixture of diastereomers, by reacting 16 with thionyl chloride. The production of new ring systems was achieved by subjecting 14 to one-pot dihydroxylation and oxidative cleavage methodology developed by Nicolaou [29] using (diacetoxyiodo)benzene, followed by reductive amination conditions. The use of dimethylamine enables the synthesis of the highly functionalized cyclohexene 23; however, more interesting heterocyclic scaffolds were accessed when primary amines were utilized, as a consequence of double reductive amination reactions. Thus, 6–6 fused ring frameworks with varied appendage diversity were obtained ( Fig. 2 , compounds 24–31 ). We observed that the reducing agent sodium triacetoxyborohydride was essential for this process, to selectively reduce the imines formed in the reaction in the presence of the aldehyde functionality. The crystal structure of 31 confirmed the expected relative stereochemistry, which had been maintained throughout this three-step, one-pot process. To further increase the diversity of the library, the dialdehyde obtained via the dihydroxylation/oxidative cleavage of 14 described above was selectively reduced to the corresponding diol and spontaneously cyclized through a ring closing transesterification reaction, yielding the novel lactone scaffold 32 in just one synthetic step. Building block 14 was viewed as a perfect substrate for molecular decoration and adornment in transition metal-catalyzed reactions. The electron-neutral alkene was amenable to ring opening/cross metathesis with terminal olefins, providing newly functionalized cyclohexene structures 33–35 . On the other hand, the ortho -bromo aryl substituent present in 14 provided a functional handle for cross-coupling reactions, introducing appendage diversity around the core scaffold. A series of Suzuki couplings to form new biaryl bonds were also performed. Although the yields for this process were poor, predominantly due to proto-debromination and the formation of compound 13 , sufficient material for biological evaluation was in hand; thus, we decided to forgo optimization of this process at that stage. In total, a library of 35 compounds with 10 distinct molecular scaffolds was synthesized ( Supplementary Fig. 2 ), comprising complex fused ring systems of varying size and a multiplicity of stereocenters. Cheminformatic analysis To computationally assess its structural diversity, we carried out a comparative statistical analysis of a set of molecular descriptors for our DOS library and two reference compound collections, comprising 40 top-selling brand-name drugs and 60 diverse natural products [30] , [31] . Principal component analysis (PCA) utilizes a defined set of molecular descriptors, such as physicochemical properties, to represent each component compound as a vector in n -dimensional space. The n -dimensional vectors can then be reduced to two-dimensional vectors by an orthogonal transformation, and re-plotted as a scatter plot, thereby providing an illustrative representation of the diversity of the compound collection. Fifteen physicochemical properties ( Supplementary Table 14 ) of the compounds were analysed using the molecular operating environment (MOE) software. The first three principal components account for 87% of the dataset variance and are represented in 2D plots ( Fig. 3a–c and Supplementary Table 15 ). As seen in Fig. 3a–c , our DOS library overlaps considerably with the chemical space explored by the top-selling drugs, indicating the potential drug-likeness of the library and possibly intimating that it should access biologically relevant areas of the chemical space. Examination of the component loadings ( Supplementary Table 16 ) shows that increases in the ring count and number of nitrogen and oxygen atoms shift molecules in the positive direction along the PC1 axes, whereas molecules with high hydrophobicity and ring count are driven in the positive direction along the PC2 axes. Important contributors to the variance in PC3 are the nitrogen atom, the aromatic atom and the ring count, an increase in all of which leads to a positive shift along the PC3 axes. These suggest that ring count is an important property contributing to the overlap between our DOS compounds and the drug library. 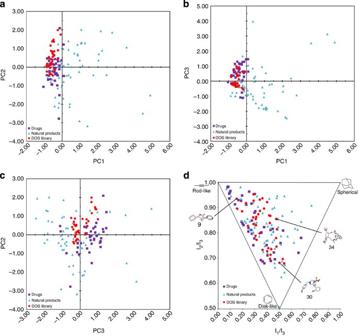Figure 3: Comparative PCA and PMI plots. Thirty-five DOS library compounds (red), 40 top-selling brand-name drugs (purple) and 60 diverse-natural products (light blue) were used; (a) PCA plot of PC1 versus PC2; (b) PCA plot of PC1 versus PC3; (c) PCA plot of PC3 versus PC2; (d) PMI plot illustrating the molecular shape diversity of the DOS library and lowest-energy conformations of three representative DOS library members. Figure 3: Comparative PCA and PMI plots. Thirty-five DOS library compounds (red), 40 top-selling brand-name drugs (purple) and 60 diverse-natural products (light blue) were used; ( a ) PCA plot of PC1 versus PC2; ( b ) PCA plot of PC1 versus PC3; ( c ) PCA plot of PC3 versus PC2; ( d ) PMI plot illustrating the molecular shape diversity of the DOS library and lowest-energy conformations of three representative DOS library members. Full size image We also compared the degree of shape diversity in our DOS library with the two reference sets of compounds. Based on the lowest-energy conformations of the compounds, normalized ratios of principal moment of inertia (PMI) were calculated and plotted on a triangular graph [32] . The PMI plot obtained ( Fig. 3d ) illustrates the shape diversity of the compounds, with its vertices representing the three extremes of molecular shape (rod, disc and sphere). The drug reference set predominantly contains rod-like shapes with some disc-like character, while the natural products exhibit considerably higher shape diversity. A very good level of shape diversity was achieved by the DOS library. We performed the Kolmogorov–Smirnov test to evaluate whether there is a significant difference between the distances of the vertices to the drugs and DOS library compounds on the PMI plot [33] . The results are not significant for distances to the disc corner ( P =0.217). However, the two libraries are significantly different in terms of distances to the other two canonical PMI shapes, with the drugs tending towards the rod corner ( P =0.027) and the DOS compounds tending towards the spherical corner ( P =0.002). This suggests that the DOS compounds contain scaffolds that are drug-like but are more spherical and three-dimensional in character than the drugs. This is particularly important, as the lack of three-dimensionality and low sp 3 carbon content is considered to be one of the main reasons why combinatorial screening collections fail to deliver hits against challenging targets such as protein–protein interactions or protein–DNA interactions [34] . Biological evaluation Antimitotic compounds are already used clinically, and this target class still holds great promise for anticancer therapy. However, resistance and administration problems have increased the requirement for new therapies [22] , [23] . One avenue to identify an antimitotic compound is by conducting a phenotypic screen for mitotic arrest. Therefore we focused our attention on a high-content screen using automated microscopy [35] , [36] . The screen was performed using U2OS osteosarcoma cells, which were incubated for 20 h with all of the library compounds, stained for the mitotic marker phospho-histone H3 and imaged on a Cellomics Arrayscan high-content microscope. Image analysis allowed us to detect the percentage of cells arrested in mitosis following compound treatment. The assay utilized nocodazole as a positive control and had a Z factor of 0.77, indicating a robust assay, particularly for a phenotypic screen ( Supplementary Fig. 3 ) [37] . All compounds were soluble at the assay concentration (50 μM), and most compounds re-screened were soluble up to 100 μM. It was encouraging to see that two molecules ( 37 and 38 ) from the original library showed mitotic arrest, with EC 50 values in the single-digit micromolar range ( Table 1 ). This is particularly significant as the library was not biased towards a particular type of target class. An additional advantage of the high-content screening approach is that one is able to identify compounds that perturb cell function without affecting the primary assay read-out. For example, we were able to identify two compounds ( 24 and 26 ) that caused a decrease in the cell viability with GI 50 ’s of 21 and 14 μM, respectively ( Supplementary Fig. 4 ), which did not induce a mitotic arrest. While we do not know the targets of these molecules, their identification is a further testament to the ability of DOS to produce potentially useful scaffolds. Table 1 Mitotic arrest EC 50 and growth inhibition IC 50 values in U2OS cells for hit compounds. Full size table Analogue synthesis In the mitotic index assay, the most potent compound ( 38 ) from the primary screen induced a marked (35–40%) mitotic arrest, which resulted in tumor cell death in a 72 h cell viability assay ( Table 1 ). Encouraged by this promising result, we sought a synthetic route that was higher yielding for analogue synthesis. It was envisaged that reducing the electron-neutral double bond would reduce the risk of side reactions in the subsequent Suzuki coupling. Moreover, biological evaluation of the reduced products would provide some structural–activity relationship information about the chemotype as well as reduce the possibility of further biochemical reactions. A new synthetic route to the reduced products was devised ( Fig. 4 ) to achieve the desired bicyclo[3.2.1]octene. Diimide reduction of intermediate 14 followed by Suzuki coupling with the appropriate boronic acids provided the desired compounds 40 and 41 in good yield. Both analogues gave a mitotic arrest in U2OS cells. In fact, comparing compound 38 with its partially saturated analogue 41 we observed a two-fold increase in potency. Treatment with 40 and 41 also resulted in growth inhibition in the low micromolar range over a period of 72 h ( Table 1 ). Given that all compounds were produced as racemates, we predicted that the antimitotic activity was likely to reside in just one of the enantiomers. Separation of both the enantiomers of dosabulin by preparative chiral HPLC and subsequent re-testing revealed that all the activity resided in the (1R,4S,5S) - enantiomer, which will henceforth be referred to as (S) - 41 ( Table 1 and Fig. 5a–c ). In fact, this enabled the use of the (R)- enantiomer as a negative control. We were then able to show that (S)- 41 treated cells died through apoptosis ( Supplementary Fig. 5 ) [38] , while cells treated with (R)- 41 did not. At this stage, we focused our attention on identifying the mechanism of action of these compounds. 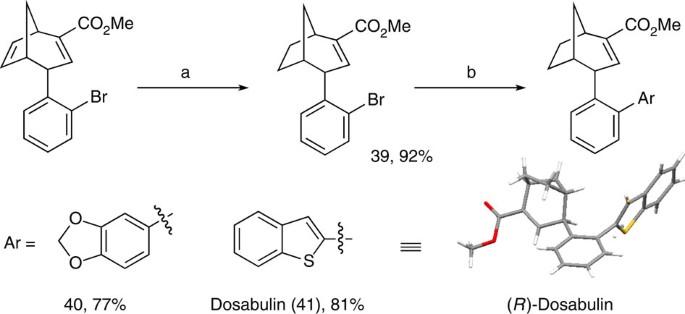Figure 4: Synthetic route to new analogues of antimitotic compounds. (a) CuCl2, hydrazine hydrate, EtOH; (b) ArB(OH)2, Pd(PPh3)4(5 mol%), 2N K2CO3, dioxane, 120 °C, μW. Figure 4: Synthetic route to new analogues of antimitotic compounds. (a) CuCl 2 , hydrazine hydrate, EtOH; (b) ArB(OH) 2 , Pd(PPh 3 ) 4 (5 mol%), 2N K 2 CO 3 , dioxane, 120 °C, μW. 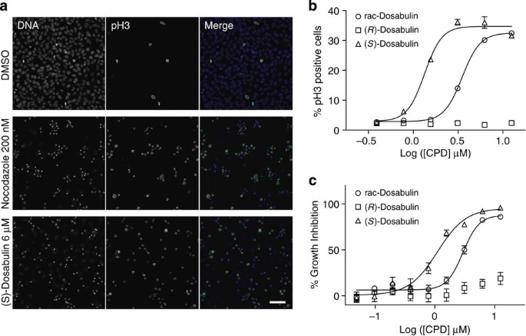Figure 5: Biological screening results of the DOS library. (a) Representative image output from the phenotypic screen, highlighting the increase in mitotic cells for those treated with the positive control nocodazole and(S)-dosabulin. U2OS cells were stained with Hoechst (blue) and a phospho-Histone H3 (pH3) antibody (green). Data were collected on a cellomics arrayscan high-content microscope with a 20x planfluor objective; scale bar: 70 μm; (b) representative mitotic index assay data in U2OS cells for racemic dosabulin and its purified enantiomers. Data points are mean±s.e.m. of an experiment conducted in triplicate. CPD=compound; (c) Growth inhibition curves in U2OS cells assessed by sulforhodamine B assay for dosabulin and its purified enantiomers. Cells were treated with compounds for 72 h, before fixing and treating with the protein dye. Data points are mean±s.e.m. of an experiment conducted in triplicate. Full size image Figure 5: Biological screening results of the DOS library. ( a ) Representative image output from the phenotypic screen, highlighting the increase in mitotic cells for those treated with the positive control nocodazole and (S) -dosabulin. U2OS cells were stained with Hoechst (blue) and a phospho-Histone H3 (pH3) antibody (green). Data were collected on a cellomics arrayscan high-content microscope with a 20x planfluor objective; scale bar: 70 μm; ( b ) representative mitotic index assay data in U2OS cells for racemic dosabulin and its purified enantiomers. Data points are mean±s.e.m. of an experiment conducted in triplicate. CPD=compound; ( c ) Growth inhibition curves in U2OS cells assessed by sulforhodamine B assay for dosabulin and its purified enantiomers. Cells were treated with compounds for 72 h, before fixing and treating with the protein dye. Data points are mean±s.e.m. of an experiment conducted in triplicate. Full size image Target identification Identification of the targets from a phenotypic screen can often be the rate-limiting step [39] . However, careful observation of the phenotype may sometimes offer clues as to what the target may be, allowing more informed experiments to be conducted [40] . Confocal microscopy was used to look at the key mitotic protein, tubulin, for this purpose. This revealed that the tubulin network was heavily disrupted on treatment with (S) - 41 compared to the DMSO control, which suggested that the compound may be targeting tubulin itself ( Fig. 6a , Supplementary Fig. 6 ). This phenotype was recapitulated by nocodazole, a known tubulin depolymerizer. This result was not altogether unexpected, given that several clinically used antimitotics target tubulin polymerization dynamics [41] . Using an in vitro tubulin polymerization assay it was established that (S)- 41 acts as a tubulin-depolymerizing agent [42] , similar to our positive control nocodazole ( Fig. 6b ). This compound was subsequently termed ‘dosabulin’. The inactive (R)- enantiomer did not show any tubulin depolymerization ability. It is widely accepted that several small-molecule binding sites exist on tubulin [43] . For example, vinblastine binds the β-tubulin subunit, while colchicine binds at the α/β interface. Additional compounds targeting tubulin dynamics exist, for which the binding site has yet to be fully elucidated, such as noscapine and peloruside. To establish whether (S)- dosabulin is bound in either of the established tubulin binding sites that cause depolymerization, two in vitro fluorescence-based assays monitoring the displacement of colchicine or vinblastine from tubulin by (S)- dosabulin were used ( Fig. 6c,d ). To monitor binding at the vinblastine site, a fluorescence polarization (FP) assay was developed. Using commercially available fluorescently tagged vinblastine it was shown that polarization increases on tubulin binding ( Supplementary Fig. 7 ). Once the optimal tubulin concentration for a sufficiently large assay window was selected, (S)- dosabulin was screened for its ability to inhibit tubulin at this site. (S)- dosabulin did not significantly affect the binding of fluorescently labeled vinblastine to tubulin in this FP assay ( Fig. 6 c and Supplementary Fig. 8 ). To determine whether (S)- dosabulin was able to bind in the colchicine site, the change in intrinsic colchicine fluorescence when bound to tubulin was measured. A time-course experiment was carried out to observe whether (S)- dosabulin was able to displace colchicine from tubulin ( Supplementary Fig. 9 ). In fact, treatment with (S) -dosabulin resulted in a time- and dose-dependent inhibition. However, incomplete inhibition was seen compared to nocodazole ( Fig. 6d ). This suggests that (S)- dosabulin may not directly displace colchicine, but rather bind to a site vicinal or allosteric to it, resulting in a decrease of its binding affinity for tubulin. 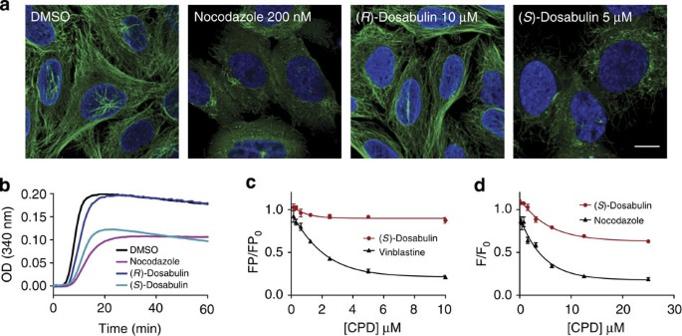Figure 6: Target identification of dosabulin. (a) Confocal microscopy in U2OS cells of both enantiomers of dosabulin show that the (S)-enantiomer disrupts the tubulin network in interphase cells, similarly to nocodazole, whilst the (R)-enantiomer does not. U2OS cells were stained with DAPI (blue) and an α-tubulin specific antibody (green). Scale bar: 15 μm; (b)in vitrotubulin polymerization data shows that (S)-dosabulin causes a decrease in tubulin polymerization, confirming this as a mechanism of action. Porcine brain tubulin (3 mg ml−1) kept at 4 °C was incubated with test compounds for 60 min at 37 °C. Compound concentrations: (S)-dosabulin and (R)-dosabulin used at 20 μM, nocodazole at 5 μM. OD=optical density; (c) fluorescence polarization (FP) data using FL-BODIPY-Vinblastine (2 μM) as a tracer shows that (S)-dosabulin does not bind tubulin in the vinblastine site. FP values were normalized to the DMSO control and data points are mean±s.e.m. of an experiment conducted in triplicate (ex/em wavelengths 485/520 nm). CPD=compound; (d) fluorescence intensity (F) measurements using colchicine show that (S)-dosabulin (red) causes a dose-dependent decrease in fluorescence without completely inhibiting the interaction, and thus is likely to bind in the vicinity or allosterically to colchicine.F-values were normalized to the DMSO control and data points are mean±s.e.m. of an experiment conducted in triplicate (ex/em wavelengths 365/435 nm). Figure 6: Target identification of dosabulin. ( a ) Confocal microscopy in U2OS cells of both enantiomers of dosabulin show that the ( S )-enantiomer disrupts the tubulin network in interphase cells, similarly to nocodazole, whilst the ( R )-enantiomer does not. U2OS cells were stained with DAPI (blue) and an α-tubulin specific antibody (green). Scale bar: 15 μm; ( b ) in vitro tubulin polymerization data shows that ( S )-dosabulin causes a decrease in tubulin polymerization, confirming this as a mechanism of action. Porcine brain tubulin (3 mg ml −1 ) kept at 4 °C was incubated with test compounds for 60 min at 37 °C. Compound concentrations: ( S )-dosabulin and ( R )-dosabulin used at 20 μM, nocodazole at 5 μM. OD=optical density; ( c ) fluorescence polarization (FP) data using FL-BODIPY-Vinblastine (2 μM) as a tracer shows that ( S )-dosabulin does not bind tubulin in the vinblastine site. FP values were normalized to the DMSO control and data points are mean±s.e.m. of an experiment conducted in triplicate (ex/em wavelengths 485/520 nm). CPD=compound; ( d ) fluorescence intensity (F) measurements using colchicine show that ( S )-dosabulin (red) causes a dose-dependent decrease in fluorescence without completely inhibiting the interaction, and thus is likely to bind in the vicinity or allosterically to colchicine. F -values were normalized to the DMSO control and data points are mean±s.e.m. of an experiment conducted in triplicate (ex/em wavelengths 365/435 nm). Full size image In this study, we report the synthesis and biological evaluation of a DOS library constructed using the rhodium (II)-catalyzed carbenoid chemistry to access key pluripotent intermediates. A total of 35 complex and structurally diverse compounds were synthesized. Biological screening of this collection in a high-content microscopy-based approach revealed two compounds that arrested cells in mitosis. Following some structural modifications we identified dosabulin, a novel small molecule that arrested cells in mitosis by depolymerizing microtubules. Dosabulin causes a dose-dependent displacement of colchicine from tubulin; however no complete disruption of the interaction is observed. This suggests that it binds in a site in the vicinity of, or allosteric to, colchicine. (S) -dosabulin causes cell death by apoptosis in U2OS osteosarcoma cells at sub-micromolar concentrations. With new tubulin-binding compounds such as eribulin recently being approved [44] , and existing therapies suffering from administration and resistance problems [22] , new antimitotics targeting tubulin are required [23] . We hope that dosabulin and related studies may spur new drug discovery efforts in this field. To further assess the utility of this library, further biological screens for antibacterial activity and the inhibition of selected protein–protein interactions are ongoing. This work validates DOS in combination with phenotypic screening as an effective strategy for the identification of new biologically relevant chemical entities. Adoption of this approach on a wide scale is likely to prove fruitful in the context of chemical genetics and drug discovery. Chemical synthesis Compounds were synthesized according to procedures specified in Supplementary Note 1 and Supplementary Methods . X-ray crystallographic data and images are reported in Supplementary Figs 10–12 and Supplementary Tables 1–13 . For 1 H and 13 C NMR spectra of compounds reported see Supplementary Figs 13–45 . Principal component analysis PCA was carried out using the MOE software package [45] . A total of 15 physicochemical properties ( Supplementary Table 14 ) were obtained for established reference sets of 40 top-selling brand-name drugs and 60 diverse natural products and 36 DOS library members [30] . The summary of the contribution of each principal component is shown in Supplementary Table 15 and the component loadings are shown in Supplementary Table 16 . The first three principal components account for 86.9% of the variance in the dataset, and were used to generate Fig. 3a–c . PMI calculations We compared the molecular shape diversity of our DOS library with the reference sets of 100 compounds used in the PCA. The stochastic conformational search algorithm in the MOE software package was used to generate 3D conformers for each compound. The MMFF94x force field was used with the generalized Born solvation model for the minimizations. Sampling and minimization parameters were implemented as follows: stochastic search limit: 7, refinement conformation limit: 300, stochastic search failure limit: 100, stochastic search iteration limit: 1,000, energy minimization iteration limit: 200 and energy minimization gradient test: 0.01. Only the conformer with the lowest energy was retained for PMI calculations in each conformational sampling run. Normalized PMI ratios ( I 1 / I 3 and I 2 / I 3 ) of these conformers were obtained from MOE and then plotted on a triangular graph, with the coordinates (0,1), (0.5,0.5) and (1,1) representing a perfect rod, disc and sphere, respectively ( Fig. 3d ). High-content analysis—mitotic index HCA was performed using an Arrayscan II HCS reader and integrated software from Cellomics. U2OS osteosarcoma cells (ATCC) were seeded in a NUNC clear flat-bottomed 96-well plate at 10,000 per well in a total of 100 μl. They were incubated at 37 °C overnight. Cells were then treated with compounds (25 μl) to give the appropriate concentration. Cells were then incubated at 37 °C for 20 h. In total 50 μl 12.5% formaldehyde was added to each well. This was incubated at RT for 10 min, before the formaldehyde was gently removed. A total of 100 μl per well permeabilization buffer (PB, contains PBS+0.1% Triton X-100), was then added to each well, incubating for 10 min. PB was removed and wells were washed with 100 μl per well blocking buffer (BB, contains PBS+1% BSA). The BB was removed and 50 μl per well of primary-antibody solution (anti-pH3 (S10), Abcam, ab5176, 1:2,000) was added. Plates were incubated for 1 h at room temperature. The antibody was removed and wells washed with 2 × 100 μl per well BB. The BB was removed and 50 μl per well of secondary-antibody solution containing Hoechst (Invitrogen, H3570, 1:2,500) and AlexaFluor-488 Goat anti-rabbit IgG (Invitrogen, A11034) was added. Plates were incubated at room temperature for 1 h in the dark. Secondary-antibody solution was removed and plates washed with 2 × 100 μl BB. The BB was then removed and 100 μl PBS/well were added. The plates were sealed with opaque film and images taken on a 20 × 0.4 NA objective. Data were analysed on Cellomics Arrayscan software using the Target Activation v4 protocol. Critical output features are: ValidObjectCount and %Responder_AvgIntenCh2. EC 50 data were calculated using Prism (Graphpad) and are an average of three independent experiments conducted in triplicate. Sulforhodamine B colorimetric assay for cytotoxicity This assay was conducted according to literarure procedure [46] . U2OS cells were seeded at 4,000 cells per well in 180 μl and incubated for 20 h at 37 °C. Compounds were then added in 20 μl to give the desired concentrations. After incubation for 72 h at 37 °C the medium was removed by aspiration and 100 μl of 1% TCA solution was added. This was incubated for 1 h and then removed. The plates were washed four times with tap water and the plates were allowed to air dry at room temperature. A total of 100 μl of a 0.057% wt by vol solution of sulforhodamine B (Sigma Aldrich) were added to each well, incubating for 30 min. The plates were then washed quickly with 4 × 100 μl of acetic acid solution (1%) and then air dried. In total 200 μl of TRIS buffer (10 mM, pH 8.0) was added to each well to resolubilize the dye. The plates were then read at 510 nm on a Infinite M200 plate reader (Tecan, Austria). GI 50 data were calculated using Prism (Graphpad), and is an average of three independent experiments conducted in triplicate. Confocal microscopy In total, 200,000 U2OS cells were seeded on coverslips in 2 mL medium in a six-well plate and incubated at 37 °C overnight. Compounds were added in DMSO to the appropriate concentration and the cells were incubated for 16 h. The medium was then aspirated and the cells were then fixed in 1 ml PBS containing 4% para -formaldehyde for 10 min. Cells were permeabilized in PBS containing 0.1% Triton-X (PBS-T) for 10 min and then washed with 1 ml PBS containing 1% BSA (PBS-BSA). Tubulin was visualized using an α-tubulin antibody (1:1,000) in 500 μl for 2 h. The primary antibody was then removed and the cells were washed with 1 ml PBS-BSA three times. Alexafluor-488 conjugated goat anti-rabbit (Invitrogen, A11034) secondary antibody was then added in 500 μl PBS-BSA for 1 h. The secondary antibody was removed and cells were washed twice with PBS-BSA and once with PBS. The coverslips were mounted on slides with a mounting medium containing DAPI and imaged on a Zeiss LSM-510 confocal microscope with a 100 × objective. Tubulin in vitro polymerization assay This assay was performed according to the literature procedure [42] . Compounds were dissolved in 10 μl 1X General Tubulin buffer (PEM) containing 80 mM Na-PIPES pH 6.9, 1 mM MgCl 2 and 1 mM EGTA, and added to wells in a 96-well plate. The tubulin solution was prepared by dissolving porcine α/β-tubulin (>99% pure, Cytoskeleton, USA) in 1X General Tubulin Buffer containing 10% glycerol and 1 mM GTP. In total 100 μl of this tubulin solution (3.0 mg ml −1 ) was added to the compound solutions or the control prewarmed in the 96-well plate at 37 °C. Tubulin polymerization was monitored over 60 min by reading the increase in absorbance at 340 nm in the Infinite M200 plate reader (Tecan). Colchicine competition assay 3 μM tubulin was incubated with 3 μM colchicine (Sigma Aldrich) and the appropriate concentrations of ( S )-dosabulin or nocodazole in PEM buffer at 37 °C for a total volume of 45 μl per well in black 384-well plates (Corning). Fluorescence readings (ex/em 365/435 nm) were taken every 15 min for 1.5 h using a Infinite M200 plate reader (Tecan). Fluorescence values were normalized to the DMSO control. Vinblastine competition assay Tubulin (2 μM) and BODIPY-FL-vinblastine (2 μM, Invitrogen) in PEM buffer were incubated with different concentrations of ( S )-dosabulin or vinblastine sulphate (Alfa Aesar) for 20 min at RT in a total volume of 45 μl per well. Fluorescence polarization readings were performed in black 384-well plates using a PHERASTAR plate reader (excitation/emission wavelengths 485/520 nm). FP values were normalized to the DMSO control. Accession codes: The X-ray crystallographic coordinates for structures reported in this article have been deposited at the Cambridge Crystallographic Data Center, under deposition numbers CCDC 936205, 936206 and 936208. These data can be obtained free of charge from the Cambridge Crystallographic Data Centre via www.ccdc.cam.ac.uk/data_request/cif . How to cite this article: Ibbeson, B. M. et al. Diversity-oriented synthesis as a tool for identifying new modulators of mitosis. Nat. Commun. 5:3155 doi: 10.1038/ncomms4155 (2014).